Maspin is not required for embryonic development or tumour suppression Maspin (SERPINB5) is accepted as an important tumour suppressor lost in many cancers. Consistent with a critical role in development or differentiation maspin knockout mice die during early embryogenesis, yet clinical data conflict on the prognostic utility of maspin expression. Here to reconcile these findings we made conditional knockout mice. Surprisingly, maspin knockout embryos develop into overtly normal animals. Contrary to original reports, maspin re-expression does not inhibit tumour growth or metastasis in vivo , or influence cell migration, invasion or survival in vitro . Bioinformatic analyses reveal that maspin is not commonly under-expressed in cancer, and that perturbation of genes near maspin may in fact explain poor survival in certain patient cohorts with low maspin expression. Maspin is a non-inhibitory member of the serpin (serine protease inhibitor) superfamily and was first identified in a screen for potential tumour suppressors lost in primary human breast cancer cell lines [1] , [2] . Consistent with tumour suppressor function, re-expression of maspin in breast tumour cell lines is reported to inhibit growth, cell migration and invasion, and increase cell adhesion [3] , [4] , [5] , [6] , [7] , [8] , [9] , [10] . Maspin downregulation has also been implicated in prostate cancer progression [11] . Although there is disagreement on the clinical utility of maspin expression as a prognostic indicator, there is major interest in understanding maspin biology, particularly with respect to the development of therapeutic strategies to combat metastasis [11] . Numerous potential molecular targets of maspin have been proposed [5] , [12] , [13] , but despite extensive effort over 20 years no study has provided a description of the physiological role of maspin that explains its tumour suppressor function. Furthermore, gene-targeted mice lacking maspin die in utero [14] , consistent with a key biological function, but complicating physiological investigations. Here we describe a new line of mice lacking maspin. Surprisingly, these animals are born and develop normally, and show no overt anatomical or physiological abnormality. We also demonstrate that maspin re-expression in transformed cells fails to suppress the neoplastic or metastatic phenotype, contrary to previous studies. Our analysis of the maspin gene locus and expression patterns in cancer suggests that maspin may be a marker of changes to an adjacent gene: the tumour suppressor, Pleckstrin Homology Leucine-rich repeat Protein Phosphatase-1 ( PHLPP1 ). Maspin itself is unlikely to function as a tumour suppressor. Generation of maspin-null mice To circumvent the problem of embryonic lethality we generated mice in which the maspin gene can be conditionally deleted, in order to abrogate maspin expression in selected tissues post-natally ( Fig. 1 ). In control experiments, two independently generated conditional lines were crossed with global Cre-deleters to delete the maspin gene from all tissues and the germ-line ( Serpinb5 tm1.1Pib (flox); Fig. 1b ). 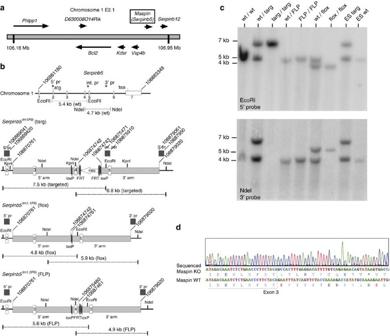Figure 1: Construction and validation of maspin knockout mice. (a) Structure of the maspin locus on mouse chromosome 1. (b) Diagrams of the maspin gene and predicted gene structure after insertion of the targeting vector (Serpinb5tm1Pib(targ)); deletion of exon 4 and the neomycin (neo) cassette after exposure to cre recombinase (Serpinb5tm1.1Pib(flox)) or deletion of the neo cassette alone after exposure to flp recombinase (Serpinb5tm1.2Pib(FLP)). Sequences cloned and used as external or internal (int.) probes (pr) are indicated. Coordinates are from the mouse genomic reference sequence GRCm38.p1 C57/BL6. (c) Validation of mouse genotypes by Southern blotting. DNA from wild type (wt) andSerpinb5tm1Pib/Serpinb5wtembryonic stem (ES) cells was used as a control. (d) Structure of maspin mRNA in ko tissue. RT–PCR product from mammary tissue was sequenced directly. Shown is a portion of the sequencing trace covering the deletion break point, with the nucleotide and inferred peptide sequences compared with the reference wt sequence below. To our surprise, inter-crosses of the resulting (±) Cre-deleted progeny yielded viable maspin −/− (knockout) animals at normal Mendelian frequency ( Supplementary Table 1 ). RNA analysis of knockout mammary tissue revealed a single maspin mRNA species carrying the predicted deletion arising from Cre-mediated recombination between loxP sites in the manipulated maspin allele ( Fig. 1d ). This shifts the reading frame and introduces a stop codon 11 residues downstream, severely truncating the protein. The predicted 133-residue mutant protein has no reactive centre loop or serpin-folding nucleus, is truncated just prior to the E-helix and would not fold if produced. In all relevant tissues examined from knockout animals, only the deleted maspin mRNA was evident ( Fig. 2a ). Figure 1: Construction and validation of maspin knockout mice. ( a ) Structure of the maspin locus on mouse chromosome 1. ( b ) Diagrams of the maspin gene and predicted gene structure after insertion of the targeting vector ( Serpinb5 tm1Pib (targ)); deletion of exon 4 and the neomycin (neo) cassette after exposure to cre recombinase ( Serpinb5 tm1.1Pib (flox)) or deletion of the neo cassette alone after exposure to flp recombinase ( Serpinb5 tm1.2Pib (FLP)). Sequences cloned and used as external or internal (int.) probes (pr) are indicated. Coordinates are from the mouse genomic reference sequence GRCm38.p1 C57/BL6. ( c ) Validation of mouse genotypes by Southern blotting. DNA from wild type (wt) and Serpinb5 tm1Pib /Serpinb5 wt embryonic stem (ES) cells was used as a control. ( d ) Structure of maspin mRNA in ko tissue. RT–PCR product from mammary tissue was sequenced directly. Shown is a portion of the sequencing trace covering the deletion break point, with the nucleotide and inferred peptide sequences compared with the reference wt sequence below. 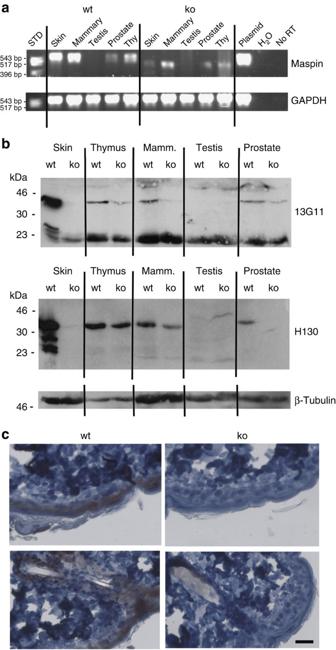Figure 2: Maspin knockout mice are ostensibly normal. (a) Comparison of maspin mRNA in adult wild-type (wt) and Cre-deleted knockout (ko) mice. Reverse transcriptase PCR analysis demonstrates products of predicted size (wt: 602 bp; ko: 455 bp), validated by DNA sequencing (seeFig. 1d). (b) ko mice do not produce maspin protein, as assessed by immunoblotting using the anti-human maspin monoclonal antibody 13G11 or rabbit anti-peptide antibody H130. Validation of these antibodies is shown inSupplementary Fig. 1. (c) Maspin ko skin lacks maspin in epidermal cells, as assessed by immunohistochemistry of samples from 8-week old mice, using 13G11. Scale bar, 30 μm. Full size image Figure 2: Maspin knockout mice are ostensibly normal. ( a ) Comparison of maspin mRNA in adult wild-type (wt) and Cre-deleted knockout (ko) mice. Reverse transcriptase PCR analysis demonstrates products of predicted size (wt: 602 bp; ko: 455 bp), validated by DNA sequencing (see Fig. 1d ). ( b ) ko mice do not produce maspin protein, as assessed by immunoblotting using the anti-human maspin monoclonal antibody 13G11 or rabbit anti-peptide antibody H130. Validation of these antibodies is shown in Supplementary Fig. 1 . ( c ) Maspin ko skin lacks maspin in epidermal cells, as assessed by immunohistochemistry of samples from 8-week old mice, using 13G11. Scale bar, 30 μm. Full size image We next performed immunoblotting and immunohistochemistry experiments to determine whether maspin protein is missing from −/− (knockout) animals ( Fig. 2b,c ). Interpretation of the immunoblotting experiments is complicated because although the mouse genome only encodes one bona fide maspin gene, it has a vastly expanded repertoire of other clade B (intracellular) serpins [15] . These are all known or predicted protease inhibitors of similar size to maspin (42 kDa), and as they are typically 40–45% identical to maspin in amino-acid sequence, they potentially represent cross-reacting targets. Only antibodies to human maspin are currently available. Of the several that we tested, two efficiently recognize mouse maspin ( Supplementary Fig. 1 ): a monoclonal (13G11) arising from our previous hybridoma screen [16] and a commercial antibody (Santa Cruz H130) reported to recognize mouse maspin [17] . In immunoblotting experiments both antibodies reported the absence of maspin in adult knockout skin ( Fig. 2b ). Notably, the pattern in other tissues was different for the two antibodies: for example, 13G11 showed the absence of maspin from knockout mammary tissue but the presence of low levels of 42 kDa species in knockout thymus and prostate, whereas H130 showed the absence of maspin from knockout prostate, little or no reduction in 42-kDa signal from knockout thymus and a reduction in 42 kDa signal in knockout mammary tissue. The simplest explanation for these results is that, as anticipated, the antibodies cross-react with other (different) mouse clade B serpins. In immunohistochemistry experiments using 13G11, maspin could not be detected in knockout epidermis ( Fig. 2c ). Thus, the DNA ( Fig. 1c ), mRNA ( Figs 1d and 2a ), immunoblotting ( Fig. 2b ) and immunohistochemistry ( Fig. 2c ) data clearly demonstrate that these knockout animals lack maspin. We next investigated whether loss of maspin resulted in any overt anatomical or reproductive phenotype. However, we found that the maspin knockout animals of both genders are indistinguishable from wild-type animals and are fertile ( Supplementary Table 1 ). Knockout dams mated to knockout males produce litters of average size and raise them normally. Taken together, our observations contradict previous findings of peri-implantation embryonic lethality (around embryonic (E) day 4.5–5.5) in maspin knockout mice [14] . Our data are however consistent with microarray analyses, which show that maspin is not expressed early in mouse embryogenesis, only appearing well after implantation, at E10.5 ( Supplementary Table 2 ). Effect of maspin re-expression on transformed cells Since these observations call into question an important aspect of maspin biology, we set out to reproduce other key experiments that originally sparked interest in this protein. Cancer cells require a microenvironment of distinct cell types to collectively enable tumour growth and progression. Such a microenvironment can only be present in vivo . Thus, in an approach similar to the original report [2] , we used two well-studied and widely used human breast cancer cell lines (MDA-MB-231 and MDA-MB-435) to investigate the effects of maspin on primary tumour growth in human breast tumour xenografts in nude mice [2] , [3] , [6] . Neither cell line expresses maspin endogenously ( Supplementary Fig. 2 ). Maspin expression was engineered in these cells by viral transduction of an expression vector containing an internal ribosomal entry site, allowing co-expression of maspin as well as dsRed, which acts as a fluorescent marker of transduced cells ( Supplementary Fig. 2a,b ). Sorted but uncloned populations of cell lines expressing maspin and dsRed (with maspin levels exceeding those in the immortalized breast epithelial cell line MCF10A ( Supplementary Fig. 2c,d )), or dsRed alone as a control, were used for subsequent in vitro and in vivo assays. Groups of eight mice were injected with 231/maspin, 231/dsRed, 435/maspin, 435/dsRed or the respective parental cell lines, and tumour growth monitored weekly. All cell lines formed tumours in 100% of injected mice ( Fig. 3a,b ). Mice implanted with MDA-MB-231 cells had faster tumour growth, with most tumours reaching a volume of 1,000 mm 3 in 4 weeks, whereas MDA-MB-435 cells took up to 8 weeks. In no case did tumours arising from cells expressing maspin show retarded growth rates ( Fig. 3a,b ). Immunoblot analysis revealed that maspin expression and level were maintained throughout tumour growth ( Fig. 3a,d ). Immunohistochemistry analyses further revealed that the morphology of the maspin-positive tumours did not differ from that of controls ( Fig. 3c,d ). 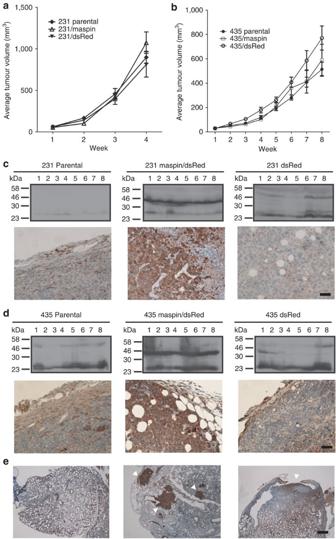Figure 3: Maspin does not affect tumour growth, size, morphology or metastasis. Balb/c nu/nu mice were implanted orthotopically with parental or transduced (maspin/dsRed or dsRed) MDA-MB-231 or MDA-MB-435 cells to generate breast tumour xenografts (six groups,n=8 per group). (a,b) Developing mammary fat pad tumours were measured twice weekly. (c) MDA-MB-231 derived tumours were examined for maspin via immunoblotting (upper panels) and immunohistochemistry (lower panels) using the monoclonal antibody 16F7. Scale bar, 50 μm. (d) MDA-MB-435-derived tumours were examined for maspin via immunoblotting (upper panels) and immunohistochemistry (lower panels) using the monoclonal antibody 16F7. Scale bar, 50 μm. (e) Micrometastatic lesions (arrowheads) were evident in all 435 xenograft types, and these lesions were positive for maspin in the 435/maspin tumours. Scale bar, 200 μm. Figure 3: Maspin does not affect tumour growth, size, morphology or metastasis. Balb/c nu/nu mice were implanted orthotopically with parental or transduced (maspin/dsRed or dsRed) MDA-MB-231 or MDA-MB-435 cells to generate breast tumour xenografts (six groups, n =8 per group). ( a , b ) Developing mammary fat pad tumours were measured twice weekly. ( c ) MDA-MB-231 derived tumours were examined for maspin via immunoblotting (upper panels) and immunohistochemistry (lower panels) using the monoclonal antibody 16F7. Scale bar, 50 μm. ( d ) MDA-MB-435-derived tumours were examined for maspin via immunoblotting (upper panels) and immunohistochemistry (lower panels) using the monoclonal antibody 16F7. Scale bar, 50 μm. ( e ) Micrometastatic lesions (arrowheads) were evident in all 435 xenograft types, and these lesions were positive for maspin in the 435/maspin tumours. Scale bar, 200 μm. Full size image We next examined the lungs of mice injected with the MDA-MB-435 set of cell lines to look for micrometastatic lesions [2] ( Fig. 3e ). Most animals presented with lesions, but there was no significant difference in the metastasis of cells expressing maspin versus those that do not. ( Supplementary Table 3 ) This contradicts the original report [2] , which showed that three out of four mice injected with maspin transfectants did not exhibit metastasis to the lung, whereas metastasis was present in both control animals. While these in vivo data suggest that maspin does not play a key role in tumour metastasis, a significant body of published in vitro data support a role for maspin in cell motility and migration. It was originally suggested that maspin is secreted from the cell and inhibits cell migration and invasion via interaction with extracellular matrix proteins [3] , [18] , [19] and β1-integrin [20] . However, these studies either followed single-cell clones of stably transfected cancer cell lines over-expressing maspin, or relied on addition of recombinant maspin to cells, with the assumption that maspin acts at the cell surface. With regards to the latter point, we have shown that maspin lacks a conventional signal peptide and cannot be secreted from the cell, suggesting strongly that it is an intracellular protein, as is the case with the majority of clade B serpins [21] . Intracellular functions for maspin have been suggested by several groups; for example, through regulating Rac and Cdc42 (refs 6 , 22 ) or the adhesion plaque [5] . Thus, we focused on maspin’s potential effect as a tumour suppressor acting from inside the cell. To study the ability of maspin to inhibit cell migration, we performed an in vitro wound-healing assay [23] , [24] comparing 231/maspin, 231/dsRed, 435/maspin, 435/dsRed cells and their respective parental cell lines. MDA-MB-435 cells generally migrated slower than MDA-MB-231 cells, but maspin expressed in either line was unable to slow cell migration ( Supplementary Fig. 3 ). We tested the ability of maspin to inhibit chemotactic migration through type I collagen, the major structural component of the extracellular matrix [25] , [26] . Maspin expression did not influence cell migration of either MDA-MB-231 or MDA-MB-435 cells ( Supplementary Fig. 4a,b ), suggesting that it does not increase adhesion and prevent migration. The ability of tumour cells to invade is a hallmark of cancer progression to malignancy. Maspin has been suggested to increase adhesion to ECM proteins and suppress invasion [2] , [3] . We tested the ability of maspin to inhibit migration through Matrigel by seeding cells expressing maspin and vector control, as well as parental cell lines on Matrigel-coated Transwells with fibroblast-conditioned medium as a chemoattractant. Maspin did not affect invasion of either MDA-MB-231 or MDA-MB-435 cell lines ( Supplementary Fig. 4c,d ). Taken together, these results suggest that maspin does not mediate its tumour-suppressive function through processes involved in cell adhesion and subsequently, cell migration. One of the fundamental traits of cancer cells is their ability to sustain proliferation. To test the involvement of maspin in cell division and colony formation, we looked at the effect of maspin on cancer cells in anchorage-dependent clone formation. Expression of maspin did not affect anchorage-dependent clone formation in MDA-MB-231 or MDA-MB-435 cell lines ( Supplementary Fig. 5a,b ). We also tested the ability of maspin to inhibit anchorage-independent clone formation, since one of the hallmarks of malignant transformation is the ability of cells to proliferate in the absence of adhesion to a subcellular matrix. Again, the re-expression of maspin in either MDA-MB-231 or MDA-MB-435 cells did not inhibit the formation of colonies ( Supplementary Fig. 5c,d ). Expression of maspin in cancer Given these data and the numerous studies that have connected differential maspin expression or cellular localization to cancer, we analysed microarray data sets to determine whether there is consistent loss or gain of maspin expression in particular cancer types. ONCOMINE [27] indicates that maspin is over-expressed in more cancer types (21 out of 313 total analyses) than under-expressed (13 out of 313 total analyses) ( Fig. 4a ). Indeed, in some cancer types, maspin can be either over-expressed or under-expressed. In comparison, PTEN , a known tumour suppressor [28] , is clearly under-expressed in cancers (under-expressed in 15/338 total analyses; over-expressed in 2). These results are consistent with observations in epidemiological/immunohistochemical studies (reviewed in ref. 29 ), where maspin has been reported to be under-expressed in some cancers but over-expressed in others [30] , [31] , [32] , [33] , [34] , [35] . 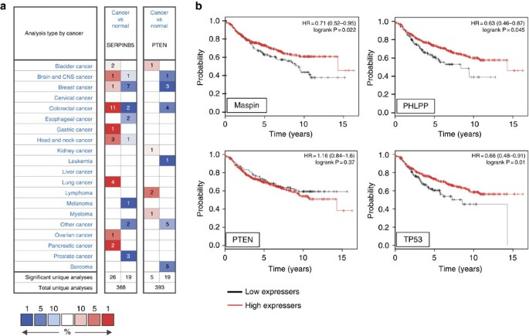Figure 4: Maspin can be over- or under-expressed in cancer. (a) Differential maspin expression between normal breast tissue and various types of cancers based on default thresholdP-value and fold changes set by Oncomine. Over-expression or under-expression in the top 1, 5 and 10% are colour-coded according to the legend. (b) Correlation between lower maspin expression (Affymetrix ID 204855_at (SERPINB5)) and poor recurrence-free survival (RFS) in some breast cancer patients. Plots were generated online using a Kaplan–Meier Plotter based on signal intensity in microarray gene expression data from patients for which recurrence-free survival data is available. Shown are plots for patients in the lower RFS quartile, and comparison toPHLPP(Affymetrix ID 212719_at (PHLPP1)),PTEN(Affymetrix ID 217492_s_at (PTEN)) andTP53(Affymetrix ID 201746_at (TP53)). Figure 4: Maspin can be over- or under-expressed in cancer. ( a ) Differential maspin expression between normal breast tissue and various types of cancers based on default threshold P -value and fold changes set by Oncomine. Over-expression or under-expression in the top 1, 5 and 10% are colour-coded according to the legend. ( b ) Correlation between lower maspin expression (Affymetrix ID 204855_at (SERPINB5)) and poor recurrence-free survival (RFS) in some breast cancer patients. Plots were generated online using a Kaplan–Meier Plotter based on signal intensity in microarray gene expression data from patients for which recurrence-free survival data is available. Shown are plots for patients in the lower RFS quartile, and comparison to PHLPP (Affymetrix ID 212719_at (PHLPP1)), PTEN (Affymetrix ID 217492_s_at (PTEN)) and TP53 (Affymetrix ID 201746_at (TP53)). Full size image Given its original description as a gene lost in breast cancer [2] , we were also particularly interested to determine whether maspin under-expression or loss correlates with malignancy and/or decreased survival in this setting. The Genome Expression Atlas (EMBL-EBI) contains two studies showing maspin under-expression in invasive ductal breast carcinoma (the most common form of breast cancer) and eight studies showing non-differential expression. To assess the external validity of maspin as a breast cancer biomarker we employed the online Kaplan–Meier Plotter, an algorithm that relates gene expression data to clinical data from 2,880 patients [36] . Using the complete data set (which comprises samples from different types and stages of breast cancer) there was no correlation between maspin expression and overall survival, recurrence-free survival or distant metastasis-free survival—in either the median, upper or lower quartiles of patients ( Table 1 ). However, if analysis is restricted to lymph node-positive (metastatic) patients, low maspin expression correlates with poorer recurrence-free survival in the lower quartile ( Fig. 4b ). A similar profile is seen with the tumour suppressor TP53 , but not with PTEN , illustrating that altered expression need not be causally linked to cancer progression and survival risk. Importantly, we noted that the maspin gene neighbour PHLPP1 ( Fig. 1a ) also shows significant under-expression in the same patient cohort ( Fig. 4b ). Table 1 The association between maspin expression and patient survival in breast cancer. Full size table Why are our findings in such dramatic contrast to others? We note that the original maspin knockout animals retain a conventional neomycin selection cassette (neo-insert) in the targeted maspin gene. By contrast, the corresponding transcriptional unit has been removed in our animals ( Fig. 1b,c ). The presence of the neo-insert can deleteriously influence expression of neighbouring genes in genetically modified animals [37] , [38] , [39] , [40] , [41] ; so, we suggest that adventitious effects of this unit may have disrupted embryonic development of the original maspin knockout mice. Related to this point, the maspin locus is conserved between mouse and human, and contains at least two genes with documented effects on cell survival: B-cell lymphoma 2 ( Bcl2 )) and PHLPP1 ( Fig. 1a ; refs 42 , 43 ). An explanation for our failure to reproduce findings that maspin re-expression modifies the transformed phenotype is that we used viral transduction as a method of gene transfer [44] , [45] . This approach eliminates the need for single cell cloning, which may select cells with different characteristics to the uncloned parental population. By contrast, most research on maspin as a tumour suppressor has been based on the analysis of limited numbers of single cell clones of MDA-MB-231 or MDA-MB-435 cells engineered to express maspin [2] , [46] ). We suggest that data obtained from such experiments may reflect clonal artefacts rather than actual maspin function. The maspin neighbour, PHLPP1 , has key characteristics of a tumour suppressor. PHLPP1 encodes a protein phosphatase that terminates signalling by pro-survival kinases via Akt inactivation, thereby promoting apoptosis. It is deleted in many cancers in which maspin has been implicated (including breast and prostate), and increased prostate intraepithelial neoplasia is observed in PHLPP1 knockout mice when combined with PTEN hemizygosity [47] . Furthermore, and in contrast to our results with maspin, PHLPP1 over-expression in cell lines derived from a variety of cancer types decreases colony formation and growth in vitro , and tumour growth in vivo . Hence, a simple explanation for the repeated failure of the field to consistently and convincingly link maspin to tumour cell biology is that maspin downregulation via chromosomal deletion or epigenetic alterations is an occasional bystander effect of selection for PHLPP1 under-expression during cancer progression. Supporting this view is the fact that no mutations in the maspin gene itself have been associated with tumours, unlike TP53 or PTEN . Phenotypic change in cancer cells lines treated with demethylation agents that has been associated with re-expression of maspin [11] can be explained by concomitant re-expression of PHLPP1. In conclusion, we have disproved the hypothesis that maspin is essential for embryonic development and life. Further, using the same cell lines and similar approaches as others, we have demonstrated that in our hands maspin does not inhibit primary tumour growth or metastasis in vivo , or cell migration, invasion and clone formation in vitro . Taken with our insight that it may be a prognostic indicator that actually reflects PHLPP1 status, we conclude that maspin is unlikely to function as a tumour suppressor. Generation and validation of maspin knockout mice The targeting vector and probes were designed and constructed by the Gene Recombineering Facility of the Australian Regenerative Medicine Institute (Monash University). The vector was built by recombination-mediated genetic engineering [48] using the bacterial artificial chromosome (BAC) clone RP23-137D2 as a source of Serpinb5 DNA. This vector ( Fig. 1b ) comprised a neomycin transcriptional unit flanked by flippase (Flp) recognition target (FRT) elements placed in intron 4. A loxP element was placed in the same intron immediately downstream of the neomycin cassette, while an upstream loxP element was placed in intron 3. A second transcriptional unit encoding Diptheria toxin A chain (DTA) was placed outside the Serpinb5 sequences to provide negative selection in transfected ES cells [49] . In brief, a zeocin selectable marker flanked by 50 bp Serpinb5 sequences (ends of 5′ and 3′ homology arms) was constructed and inserted into pDTA-TKIII (ref. 50 ). This plasmid was linearized and electroporated into E.coli containing the BAC to capture the Serpinb5 gene-targeting fragment into the pDTA vector via homologous recombination, which results in loss of the zeocin gene. Again via homologous recombination, a loxP-neomycin-loxP cassette flanked by 50 bp sequences homologous to intron 3 of Serpinb5 was inserted into the pDTA-targeting vector. A Cre recombinase deletion step in E.coli was then performed to remove the neomycin cassette, leaving a single loxP site upstream of the exon. Finally, a FRT-PGK-neo-FRT-loxP cassette [50] guided by 50-bp Serpinb5 flanks was inserted in intron 4. The final construct and probes were sequenced overall junctions. The Serpinb5 knockout mice were produced by the Monash Gene Targeting Facility and were housed in specific-pathogen-free animal facilities. Bruce 4 C57BL/6-derived embryonic stem (ES) cells were transfected as described [51] , [52] with the linearized targeting construct, selected in G418, and 400 resulting clones analysed by Southern blotting with the 5′ external probe on Eco RI-cleaved genomic DNA (wt 5.4 kb; KO 7.5 kb) and the 3′ external probe on Nde I-cleaved DNA (wt 4.7 kb; KO 6.8 kb). Fifteen clones were identified as homologous recombinants. Eight of these clones were re-confirmed as positive by analysis of SpeI-digested DNA with the 5′ external probe (wt 14.5 kb; KO 10.5 kb) and NdeI-digested DNA using the 3′ external probe. The 8 positive clones were also analysed on EcoRI-cleaved or BsrGI-cleaved DNA using the internal probe. Six out of 8 clones were shown to have integrated one copy of the construct and did not show off-target events. DNA from two correctly targeted clones containing the Serpinb5 tm1Pib allele (MGI:5484763) were injected into BALB/c blastocysts to generate chimeric mice, which were crossed to C57BL/6 Cre-deleter transgenic mice (Tg(CMV-cre)1Cgn [53] ) to remove exon 4 and the neomycin cassette from the targeted allele and produce two lines of animals carrying the Serpinb5 tm1.1Pib mutation (MGI:5484764). In parallel, chimeric mice were crossed to C57BL/6 Flp-deleter transgenic mice [54] to remove the neomycin cassette only ( Serpinb5 tm1.2Pib (MGI:5484765)). Floxed mice heterozygous for the Serpinb5 tm1.1Pib mutation were inter-crossed to generate mice of all three genotypes. To genotype mice, DNA from tail biopsies taken at 11 days of age was analysed by PCR using the primers listed in Supplementary Table 4 . PCR for the Serpinb5 -targeted mutation used oligonucleotides PB1604 and PB1618, 200 μm dNTPs, 25 pmol each primer, 2 mM MgCl 2 and Taq polymerase, at 95 °C for 1 min, 58 °C for 1 min, 72 °C for 1 min, over 35 cycles. The PCR for the Serpinb5 tm1Pib -targeted mutation amplified a 360-bp product from the wt allele and a 450-bp product from the targeted allele. Offspring from mice heterozygous for the targeted mutation crossed to Cre-deleter mice, and subsequent progeny were similarly genotyped by PCR, but required two separate reactions. PB1668 and PB1671 amplified a 460-bp product from the wt allele and PB1668 and PB1670 amplified a 450-bp product from the Serpinb5 tm1.1Pib mutant allele. Final genotype validation of targeted, floxed and flped mice involved Southern analysis of spleen genomic DNA using Eco I cleavage and the 5′ external probe, Nde I cleavage and the 3′ external probe ( Fig. 1c ), and Kpn I cleavage and the internal probe. To assess mRNA production in tissues, mRNA was isolated from skin, mammary glands, testis, prostate and thymus. Tissue samples were homogenized in 1 ml of Trizol. Following RNA extraction and DNase treatment (Promega), 3 μg of RNA per sample was reverse transcribed using SuperScript III First-Strand Synthesis System. PCR primers were designed to anneal to exon 2 and exon 6 of maspin cDNA (PB1687, PB1688) or GAPDH cDNA ( Supplementary Table 4 ). Cycling conditions for maspin primers were 95 °C for 30 s, 58 °C for 30 s, 72 °C for 30 s over 35 cycles. GAPDH primers were used at denature 95 °C for 30 s, 55 °C for 30 s, 72 °C for 1 min over 30 cycles. WT (602 bp) and KO (455 bp) products were cut from a 1% agarose gel and purified (UltraClean 15 UltraBIND). The DNA was sequenced with forward (PB1688) and reverse (PB1687) maspin primers. Organ and tissue isolation and analysis Histopathological assessments of two male and two female 6-week-old mice and clinical haematological analysis of one male and one female mouse were performed via the Australian Phenomics Network ( http://www.australianphenomics.org.au/ ). The following organs were examined for macromorphological abnormalities: testes, epididymes, seminal vesicles, prostate glands, penis, preputial gland, mammary tissue, ovaries, oviducts, uterus, cervix, vagina, clitoral gland, bladder, liver, gall bladder, stomach, duodenum, jejunum, ileum, caecum, colon, mesenteric lymph node, spleen, pancreas, kidney, adrenal glands, salivary glands and regional lymph nodes, thyroids, trachea, lungs, thymus, heart, skin, tail, eyes, harderian glands, brain, spinal cord and hind leg. For haematological analysis blood samples from 7-week-old mice mice collected into EDTA were run on the Advia 2120 Haematology system, which gives a red blood cell count (with indices), platelet count, and a white blood cell differential by size, granularity and peroxidase absorption. Cell culture MDA-MB-231 (231) and MDA-MB-435 (435) cells were maintained in DME supplemented with 10% ( v / v ) FCS, 50 U of penicillin per ml, 50 μg of streptomycin per ml and 2 mM glutamine. HEK-293T cells were also cultured in DME supplemented with 10% ( v / v ) FCS, 50 U of penicillin per ml, 50 μg of streptomycin per ml and 2 mM glutamine. Plasmids For the expression of maspin in 231 and 435 cells, a maspin cDNA was amplified by PCR using the oligonucleotide primers 5′-GGGAGATCTCATGGATGCCCTGCAACTAGC-3′ and 5′-CCCGCGGTTAAGGAGAACAGAATTTGCC-3′ and Taq DNA polymerase (New England Biolabs) for 25 cycles of 95 °C for 45 s, 55 °C for 45 s and 72 °C for 90 s. The resulting 1.15-kb product was cloned into pCR-Blunt (Invitrogen), confirmed to be maspin by sequencing, then released and purified as an Eco RI– Eco RI fragment. Blunt ends were then generated by Klenow fill-in, and fragments cloned in-frame in pLoxIRESdsRed digested with Sma I and de-phosphorylated using TSAP thermosensitive alkaline phosphatase (Promega). CaPO 4 transfection of HEK-293T cells Ten 100-mm dishes of HEK-293T cells seeded at 1 × 10 6 cells per dish were transfected with a total of 25 μg DNA (50% pLoxIRESdsRed/maspin or pLoxIRESdsRed alone, 17.5% pMD2G (viral envelope proteins), 32.5% psPAX2 (viral packaging proteins)) and 25 μg carrier DNA in 0.1 × TE, pH 7.6 (1 mM Tris, 0.1 mM EDTA, pH 8.8) in a volume of 4.5 ml. To this, 500 μl of CaCl 2 was added, mixed well and then 5 ml 2 × HBS (280 mM NaCl, 100 mM HEPES, 1.5 mM Na 2 HPO 4 , pH 7) was added drop-wise while DNA mix was agitated gently. Flocculent precipitates were then allowed to form over 30 min in room temperature and 1 ml of the DNA/CaPO 4 mix added to each 100-mm dish of HEK-293T cells. Cells were incubated overnight, medium replaced and viral supernatant collected 24, 40, 48 and 64 h after transfection. Stable transduction of MDA-MB-231 and MDA-MB-435 cells Cells were transduced as described [55] . Briefly, 2.5 × 10 5 cells in 3.3 ml of complete growth medium was mixed with 6.7 ml of viral supernatant, and Polybrene (Sigma) added at a final concentration of 12 μg ml −1 . Cells were incubated overnight, subjected to a second round of infection using viral supernatant collected at 40 h, then viral supernatant replaced with complete growth medium on the third day. Cells were then FACS sorted to isolate dsRed-positive cells. Antibodies Mouse anti-human maspin monoclonal antibodies were raised against recombinant maspin produced in Escherichia coli [56] . Antibodies were tested for the ability to recognize mouse maspin expressed in COS cells, by immunoblotting and indirect immunofluorescence. Secondary antibody used in immunoblotting was sheep anti-mouse IgG conjugated to horseradish peroxidise (Chemicon), and secondary antibodies used in indirect immunofluorescence were goat anti-mouse IgG conjugated to Alexa Fluor 488 (Invitrogen). SDS–PAGE and immunoblot analysis Equal amount of cell lysates in NP40 lysis buffer with protease inhibitors (50 mM Tris, pH 8.0, 10 mM EDTA, 1% ( v / v ) Nonidet P40), as determined by BioRad Protein Assay according to manufacturer’s instructions, were resuspended in Laemmli sample buffer with 100 mM DTT and loaded onto a 12.5% SDS–PAGE. Samples were resolved for 1 h at 200 V and then transferred onto nitrocellulose blot for 1 h at 250 mA. Blot was then blocked in Blotto (5% ( w / v ) skim milk powder in Tris saline (20 mM Tris, 150 mM NaCl)) for 1 h at room temperature, and incubated in 1:1,000 dilution of mouse anti-maspin monoclonal antibody overnight at 4 °C with gentle rocking. Unbound primary antibodies were then washed off with Tris-Tween (Tris saline with 0.001% ( v / v ) Tween), and blot was incubated with 1:5,000 diluted sheep anti-mouse IgG conjugated to horseradish peroxidise (Chemicon) for 1 h at room temperature, after which unbound secondary antibodies were washed off with Tris-Tween. Blot was then incubated in Western Lightning Plus-ECL (PerkinElmer) according to manufacturer’s instructions, exposed to X-ray film and film developed. Indirect immunofluorescence Cell monolayers grown on 10-well microscope slides were washed in PBS containing 0.1 mM CaCl 2 and 1.0 mM MgCl 2 (PBS+), fixed in 3.7% formaldehyde in PBS+ for 20 min, quenched with 20 mM ammonium chloride and permeabilized by incubation in 0.5% Triton X-100 in PBS+ for 5 min. Antigens were detected by incubation of the cells for 30 min with 1:1,000 diluted mouse anti-maspin monoclonal antibody. After being washed with PBS+ the cells were incubated with 1:800 dilutions of Alexa 488-conjugated secondary antibodies. After 30 min cells were washed in PBS+ then mounted in MOWIOL. Wound-healing assay Cells at a density of 7.0 × 10 5 cells per ml were seeded onto each chamber of a Culture-Insert (Ibidi) in six-well plates, which were gently removed the next day to reveal a wound. Cells monolayers were then washed gently with PBS+ to clear away debris, and assayed in complete growth medium supplemented with 1 ng ml −1 Mitomycin C for 24 h. Images of cells were taken every 30 min using Leica AF6000LX Live Cell Imaging workstation and included LASAF software. The cell migration rate was calculated as the distance travelled by the cells over time by measuring the change in cell-free areas measured at specified time-points using Image J. Cell migrated into the previously cell-free area came from two directions. Thus, to calculate the distance travelled by the migrating cells, the change in cell-free area (measured as a fraction of the total image area) was multiplied by the width of the image (520 μm), then divided by 2. Migration rate was then calculated as distance (μm) travelled per hour. The mean and s.e.m were calculated and graphed using GraphPad Prism software. Collagen I chemotactic migration assay Transwells (8.0 μm, pore size 6.5 mm; Corning) were coated with Collagen I at 20 μg ml −1 in 10 mM acetic acid overnight, then air-dried and placed onto wells of a 24-well plate. Cells were trypsinized, resuspended in base DME with 0.1% ( w / v ) BSA at the density of 0.5 × 10 6 cells per ml and 100 μl of this resuspension seeded in the coated Transwell (top chamber). Fibroblast-conditioned medium (600 μl) was then added to the well of the 24-well plate (bottom chamber). Cells were allowed to migrate at 37 °C for 5 h. Each cell line was seeded in triplicate. Cells that have not migrated from the top chamber were then removed using a cotton swab, and cells that have migrated to the bottom of the membrane were fixed in methanol for 15 min at room temperature, then stained with Crystal Violet. Wells were shuffled by a technician, and returned for counting in a blinded fashion. Migration through Collagen I to the bottom of the Transwell membrane was quantified by counting five random fields. The mean and s.e.m were calculated and graphed using GraphPad Prism software. Matrigel invasion assay Matrigel invasion assays were performed as described [57] . Briefly, 8.0-μm pore size 6.5 mm Transwells (Corning) were coated with 0.125 μg μl −1 Matrigel, then air-dried and placed onto wells of a 24-well plate. Coated wells were reconstituted with base DME for 1 h before assay. Cells were trypsinized, resuspended in base DME with 0.1% ( w / v ) BSA at the density of 0.25 × 10 6 cells per ml and 100 μl of this resuspension seeded in the coated Transwell (top chamber). Fibroblast-conditioned medium (600 μl) was then added to the well of the 24-well plate (bottom chamber). Cells were allowed to migrate at 37 °C for 24 h. Each cell line was seeded in triplicate. Cells that have not migrated from the top chamber were then removed using a cotton swab, and cells that have migrated to the bottom of the membrane were fixed in methanol for 15 min at room temperature and stained with 0.2% ( w / v ) Crystal Violet in 2% ethanol. Wells were shuffled by a technician and returned for counting in a blinded fashion. Invasion through Matrigel to the bottom of the Transwell membrane was quantified by counting five random fields. The mean and s.e.m were calculated and graphed using GraphPad Prism software. Anchorage-dependent clonogenic assay Fifty cells were seeded in wells of a six-well tray and colonies allowed to form for 2 weeks. Each cell line was seeded in triplicate. Growth medium was replaced every 3 days. Once visible, colonies were fixed for 15 min at room temperature with methanol, then stained with 0.01% Crystal Violet and counted. The mean and s.e.m were calculated and graphed using GraphPad Prism software. Anchorage-independent clonogenic assay A base layer of 1% ( w / v ) agar in complete growth medium was prepared and 2 ml was laid on wells of a six-well tray. Base agar was allowed to solidify for at least 30 min. The base layer was then overlaid with 10,000 cells per well resuspended in 0.5% agar in complete growth medium. Once set, complete growth medium was then added on top of the cell-agar layer, and replaced every 3 days for 2–3 weeks. Once visible, colonies were stained with 1 ml 0.005% ( w / v ) Crystal Violet overnight and counted. The mean and s.e.m were calculated and graphed and Student’s t- test done using GraphPad Prism software. Mammary fat pad injections Forty eight female BALB/c nu/nu mice at 5–6 weeks of age were obtained from Animal Resources Centre (Australia) with ethics approval from School of Biomedical Sciences Animal Ethics Committee, Monash University (Project number: MARP/2011/040). Mice were allowed to acclimatize in pathogen-free agistment for 2 weeks before inoculation. Cells for inoculation were prepared at a density of 1.3 × 10 8 cells per ml and mixed with equal amounts of growth factor reduced Matrigel (BD Biosciences). A total of 15 μl of this cell/Matrigel suspension was injected into each mouse at the #4 mammary fat pad of Balb/c nu/nu mice. Growing primary tumours were measured twice weekly. Once tumours grew to a total volume of 1 cm 3 , mice were killed. Tumours were then dissected out, weight recorded and processed for protein analysis by western blotting and immunohistochemical analyses. The mean and s.e.m. of tumour volumes were calculated and graphed using GraphPad Prism. Analysis of lung metastasis Lungs were stained by intra-tracheal injection of 15% ( v / v ) India ink then washed in Fekete’s solution (300 ml 70% ( v / v ) ethanol, 30 ml 37% ( v / v ) formaldehyde and 5 ml glacial acetic acid), and placed in fresh Fekete’s solution overnight. Pulmonary metastases were then counted. Immunohistochemistry Skin, primary tumours or lungs were fixed in 10% ( v / v ) Formalin overnight then embedded in paraffin and 5-μm sections cut and placed onto charged slides. Sections were dewaxed and rehydrated in a gradient of ethanol/dH 2 0, then endogenous peroxidises inactivated with 3% ( v / v ) H 2 O 2 in methanol solution, and antigens retrieved by microwaving slides in TE buffer (Tris, EDTA, pH 9.0). Slides were washed in PBS containing 1% ( v / v ) Tween (PBST) and blocked with 2% BSA ( w / v ) in PBS for 10 min. For analysis of wt or knockout skin, mouse anti-maspin monoclonal antibody 13G11 (ref. 16 and Supplementary Fig. 6 ) was diluted 1:500 in 1% BSA ( w / v ) in PBS and incubated overnight on sections at room temperature. For xenotransplant analysis, mouse anti-maspin monoclonal antibody 16F7 (ref. 16 ) was diluted 1:200 in 1% BSA ( w / v ) in PBS and incubated overnight on sections at room temperature. Bound antibody was detected by biotinylated rabbit anti-mouse IgG (Rockland) at 1:200 dilution for 30 min, followed by HRP-conjugated streptavidin (Chemicon) at 1:200 dilution for 30 min and visualized using the Liquid DAB Chromogen Substrate System (DAKO, Denmark). Harris’ hematoxylin solution (Sigma-Aldrich, USA) was used as a counter-stain and slides were mounted in MOWIOL reagent. Slides were viewed under an Olympus CKX41 light microscope. How to cite this article: Teoh, S. S. Y. et al . Maspin is not required for embryonic development or tumour suppression. Nat. Commun. 5:3164 doi: 10.1038/ncomms4164 (2014).